Conformational targeting of intracellular Aβ oligomers demonstrates their pathological oligomerization inside the endoplasmic reticulum Aβ oligomers (AβOs) are crucially involved in Alzheimer’s Disease (AD). However, the lack of selective approaches for targeting these polymorphic Aβ assemblies represents a major hurdle in understanding their biosynthesis, traffic and actions in living cells. Here, we established a subcellularly localized conformational-selective interference (CSI) approach, based on the expression of a recombinant antibody fragment against AβOs in the endoplasmic reticulum (ER). By CSI, we can control extra- and intracellular pools of AβOs produced in an AD-relevant cell model, without interfering with the maturation and processing of the Aβ precursor protein. The anti-AβOs intrabody selectively intercepts critical AβO conformers in the ER, modulating their assembly and controlling their actions in pathways of cellular homeostasis and synaptic signalling. Our results demonstrate that intracellular Aβ undergoes pathological oligomerization through critical conformations formed inside the ER. This establishes intracellular AβOs as key targets for AD treatment and presents CSI as a potential targeting strategy. The proteolytic processing, misfolding and self-aggregation of several proteins are often associated with pathological conditions and conformational diseases. However, the identification, study and targeting of different conformations and multimeric states of a given protein in the complex context of subcellular compartments/microdomains of living cells remains a big challenge. A most relevant example of such a challenge is represented by the amyloid-β (Aβ) peptides, crucial players of Alzheimer’s disease (AD) pathogenesis [1] , [2] , [3] , [4] . In living cells, differently than in a test tube containing only synthetic peptides, the Aβ species are generated from the amyloid precursor protein (APP) by a complex process of regulated intramembrane proteolysis (RIP) [5] , [6] , and undergo a process of misfolding and aggregation, whose mechanism and subcellular localization(s) are still debated [7] . In particular, along the aggregation pathways, naturally occurring Aβ oligomers (AβOs) are still considered mysterious entities in terms of molecular and structural composition and activity [8] , even though they are recognized as the most neurotoxic proteinaceous forms in AD [8] , [9] . As an additional level of complexity, APP–RIP generates different proteolytic fragments and shares the secretases (both α, β and γ) with numerous different substrates [5] . Thus, the cellular biochemistry of Aβ is representative of two general mechanisms operating in living cells and organisms, namely RIP and amyloid formation (proteins enriched in cross β-sheet and prone to self-aggregation) and represents not only a pathologically relevant target, but also an ideal test case for the development of new approaches for studying these processes in cells. Conformational-sensitive antibodies are important tools for analysing amyloid assembly states and dynamics [10] . In particular, recombinant antibody fragments can be exploited as intracellular antibodies (intrabodies) for a subcellular-localized interference to block or modulate the function of target molecules [11] , [12] . In principle, if the intrabodies are intrinsically equipped with conformational-sensitive binding properties, they could be exploited for interference studies not currently feasible with nucleic acid targeting methods (that is, RNA interference or gene knockout), that can silence entire gene products (that is, APP or RIP machinery protein components) but not peculiar post-translational modification products (such as AβOs). Furthermore, even though new chemical modulators and inhibitors for APP–RIP or for Aβ assembly are intensively studied, their molecular selectivity and their precise subcellular delivery and actions remain not easy to control. In the current state of the art, while several conformation- and oligomeric-specific antibodies targeting the Alzheimer’s AβOs have been developed [8] , they are largely not exploitable for subcellular targeting and intracellular functional studies in living cells. We generated, by an in vivo intracellular selection in yeast cells, a panel of conformation-sensitive antibody fragments selectively recognizing AD-relevant AβO conformers [13] ideal for the expression (as genes) in mammalian cells, as intrabodies targeted to different subcellular compartments. Here we expressed the anti-AβO single-chain antibody fragment (scFv) A13 (ref. 13 ) as an intrabody, with the aim of intercepting AβOs at subcellular sites of their putative formation, and of attempting their functional silencing. In this way, we established a new experimental paradigm of subcellular-localized and conformational-selective interference (CSI). The intrabody-based CSI besides providing a novel approach to selectively control biologically-active AβO conformers in living cells, allows a new dissection of cellular mechanisms of AβO generation, trafficking and actions. Indeed, by exploiting CSI, we demonstrate that intracellular Aβ can oligomerize into pathological forms, through critical conformations formed inside the endoplasmic reticulum (ER). The anti-AβOs intrabody selectively intercepts critical AβO conformers and controls their ‘toxic’ assembly in the ER, without interfering with the complex processes of maturation and processing of APP. Remarkably, the pool of targeted AβO conformers are involved in the deregulation of two independent pathways of cellular homeostasis and synaptic signalling. Our overall results firmly establish the ER as the site of formation of critical Aβ conformers and validate ER-formed intracellular AβOs as a key target for AD. For these reasons, the anti-AβOs CSI can be exploitable for in vivo therapeutic applications as well as to improve our understanding of the molecular and cellular processes of AD pathogenesis, thereby uncovering new targets for drugs development. Indeed, one of the earliest events in AD pathogenesis seems to be the intraneuronal Aβ oligomerization [14] , [15] and the synaptic targeting of AβOs [3] , [16] and current studies on the intracellular Aβ generation and oligomerization do not offer yet a common and conclusive opinion, also for the lack of adequate experimental tools of study. The anti-AβO scFvA13 expressed as an intrabody in mammalian cells This study is based on scFvA13, a recombinant antibody fragment generated by a direct intracellular selection of functional intrabodies in yeast cells against the in vivo misfolded antigen Aβ [13] . The scFvA13 selectively recognizes conformational Aβ epitopes, as attested by the preferential binding in vitro to synthetic oligomeric assemblies, such as the amyloid-derived diffusible ligands (ADDLs [17] ), but not to the monomeric or fibrillar states [13] . Furthermore, the oligomeric-specific scFvA13-purified protein was characterized for its neutralizing properties against synthetic ADDLs [13] or against endogenous Aβ species [18] as well as for the recognition of pathological AβO deposits in the brain of a mouse model of familial AD (fAD) [19] and of other neurodegeneration models [20] . The conformation sensitivity of scFvA13 is accompanied by a sequence specifity for Aβ [13] , as also attested by dot blot (DB) assay ( Fig. 1a ) and enzyme-linked immunosorbent assay (ELISA) ( Supplementary Fig. 1 ), which show the lack of immunoreactivity with other proteins forming oligomers, such as α-Synuclein and lysozyme, at variance with the generic anti-oligomer A11 (ref. 21 ) ( Supplementary Fig. 1 ). 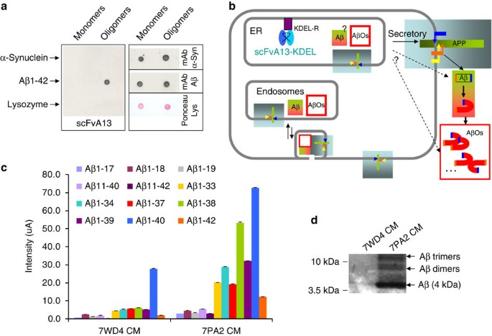Figure 1: The anti-AβOs scFvA13 exploited as intrabody in APP–RIP cell models. (a) Conformation sensitivity and sequence specificity of anti-AβOs scFvA13. Monomers and oligomers of human α-synuclein, human Aβ1-42 and lysozyme were assayed by DB with scFvA13 as primary antibody (panel on the left). The scFvA13 is revealed through its C-terminal V5 tag. As a control, the same samples were respectively analysed through a mAb anti α-synuclein (α-syn), the mAb anti-Aβ 6E10 and by Ponceau S (panels on the right). The recognition of scFvA13 is selective and specific for oligomers of human Aβ1-42, but not for other proteins, as also shown by ELISA inSupplementary Fig. 1. (b) Cartoon illustrating APP–RIP (grey–light blue-shaded box), Aβ misfolding (green–red-shaded box), Aβ oligomerization (box with a red frame) and trafficking in different (sub)cellular sites (also presumptive, indicated by the question marks) as well as the localization of intrabody scFvA13-KDEL in the ER. α-, β- and γ-secretase are represented by yellow, orange and blue arrows, respectively and Aβ misfolding by a change of a green fragment into a red hairpin. Some FAD mutations, such as the hAPPV717F brought by the APP–RIP cell model 7PA2, alter the γ-secretase cleavage determining pathological and unbalanced patterns of Aβ peptides (Supplementary Fig. 2). (c) Immunoproteomic (anti-Aβ 6E10+4G8 SELDI-TOF MS) profiles of Aβ monomers and Aβ truncated forms secreted by 7WD4 (CHO-hAPPwt) and 7PA2 (CHO-hAPPV717F) cells. The levels of Aβ fragments and monomers are significantly higher in 7PA2 CM than in 7WD4 CM. Detailed ratios (7PA2/7WD4) for each Aβ species are reported inSupplementary Table 1. Among these, the ratios for Aβ1-40 and for Aβ1-42 are 2.6 and 6.3, respectively. In addition, the fAD relevant Aβ1-42:Aβ1-40 ratio is ~\n1:15 in 7WD4 and ~\n1:6 in 7PA2. The C-terminal truncated forms (ranging from Aβ1-33 to Aβ1-42) are the most abundant species detected in 7PA2 CM (Supplementary Table 1). The histogram shows the intensity (microampere, uA) of single proteomic peaks. Mean values±s.e.m.,n=4,P<0.001, Student’st-test. (d) WB analysis (anti-Aβ 6E10) of 7PA2 and 7WD4 CM (both 15 × concentrated). Aβ and AβOs (LDS/SDS-stable Aβ dimers and trimers) are almost exclusively detected in 7PA2 CM. Figure 1: The anti-AβOs scFvA13 exploited as intrabody in APP–RIP cell models. ( a ) Conformation sensitivity and sequence specificity of anti-AβOs scFvA13. Monomers and oligomers of human α-synuclein, human Aβ1-42 and lysozyme were assayed by DB with scFvA13 as primary antibody (panel on the left). The scFvA13 is revealed through its C-terminal V5 tag. As a control, the same samples were respectively analysed through a mAb anti α-synuclein (α-syn), the mAb anti-Aβ 6E10 and by Ponceau S (panels on the right). The recognition of scFvA13 is selective and specific for oligomers of human Aβ1-42, but not for other proteins, as also shown by ELISA in Supplementary Fig. 1 . ( b ) Cartoon illustrating APP–RIP (grey–light blue-shaded box), Aβ misfolding (green–red-shaded box), Aβ oligomerization (box with a red frame) and trafficking in different (sub)cellular sites (also presumptive, indicated by the question marks) as well as the localization of intrabody scFvA13-KDEL in the ER. α-, β- and γ-secretase are represented by yellow, orange and blue arrows, respectively and Aβ misfolding by a change of a green fragment into a red hairpin. Some FAD mutations, such as the hAPPV717F brought by the APP–RIP cell model 7PA2, alter the γ-secretase cleavage determining pathological and unbalanced patterns of Aβ peptides ( Supplementary Fig. 2 ). ( c ) Immunoproteomic (anti-Aβ 6E10+4G8 SELDI-TOF MS) profiles of Aβ monomers and Aβ truncated forms secreted by 7WD4 (CHO-hAPPwt) and 7PA2 (CHO-hAPPV717F) cells. The levels of Aβ fragments and monomers are significantly higher in 7PA2 CM than in 7WD4 CM. Detailed ratios (7PA2/7WD4) for each Aβ species are reported in Supplementary Table 1 . Among these, the ratios for Aβ1-40 and for Aβ1-42 are 2.6 and 6.3, respectively. In addition, the fAD relevant Aβ1-42:Aβ1-40 ratio is ~\n1:15 in 7WD4 and ~\n1:6 in 7PA2. The C-terminal truncated forms (ranging from Aβ1-33 to Aβ1-42) are the most abundant species detected in 7PA2 CM ( Supplementary Table 1 ). The histogram shows the intensity (microampere, uA) of single proteomic peaks. Mean values±s.e.m., n =4, P <0.001, Student’s t -test. ( d ) WB analysis (anti-Aβ 6E10) of 7PA2 and 7WD4 CM (both 15 × concentrated). Aβ and AβOs (LDS/SDS-stable Aβ dimers and trimers) are almost exclusively detected in 7PA2 CM. Full size image Here, we tailored the scFvA13 for intrabody expression in subcellular compartments of living cells [12] , to target critical conformations of Aβ oligomeric assemblies naturally occurring inside cells and to intercept AβOs where they are formed in the cell. As a transmembrane protein, APP is cotranslationally inserted in the membrane of the ER, where it traffics through the other subcellular compartments of the secretory pathway; however, the role of the ER in the APP–RIP and Aβ generation, but especially in Aβ misfolding and oligomerization, remains to be deciphered ( Fig. 1b ). We exploited the scFvA13 intrabody, to ask the question as to where and when, during the APP maturation and trafficking, is Aβ formed and oligomerized, starting from the early secretory compartment. To this aim, the scFvA13 was targeted to the ER, through a C-terminal KDEL fusion allowing its ER retention and its retrieval from the cis-Golgi, through the ER-Golgi intermediate compartment [12] , [22] . In detail, the cDNA of scFvA13-KDEL was stably expressed in the 7PA2 fAD cell line [23] , [24] (CHO cells overexpressing fAD human V717F APP mutant, Supplementary Fig. 2 ), which represents a widely used model of Aβ oligomerization and the best characterized source of natural, pathologically relevant and bioactive AβOs [3] , [8] , [9] , [24] , [25] , [26] . Furthermore, the scFvA13-KDEL intrabody was expressed in CHO transfectants expressing wild-type human APP referred to as 7WD4 (ref. 23 ) ( Supplementary Fig. 2 ), which show much lower rates of Aβ production and oligomerization in comparison with 7PA2 ( Fig. 1c,d ) and in human neuroblastoma SHSY5Y cells, expressing only the endogenous APP, that show effective RIP and negligible Aβ oligomerization. Measuring Aβ and AβOs biochemical patterns in 7PA2 cells The detection of the pathologically relevant Aβ and AβOs biochemical patterns in 7PA2 cells is essential prerequisite to study the effects of the subcellular targeting of scFvA13 intrabody. An Aβ immunoproteomic analysis, based on the use of anti-Aβ (monoclonal antibody (mAb) 6E10 and 4G8) as capturing antibodies in SELDI-TOF mass spectrometry (MS) [27] , allows directly revealing the complex profile of Aβ monomers and fragments secreted by cells in the conditioned medium (CM). In this way, by comparing the 7PA2 and 7WD4 cells (respectively expressing the V717F mutant or the wild-type human APP), we measured in 7PA2 CM higher levels of secreted Aβ peptides ( Fig. 1c ) and, most importantly, a fAD-related higher Aβ1-42:Aβ1-40 ratio ( Fig. 1c , Supplementary Table 1 ). Of note, we observed an overall unbalanced proportion of carboxy- and amino-terminally truncated Aβ peptides ( Supplementary Table 1 ) in 7PA2 CM, similar to Aβ profiles in cerebrospinal fluids from human fAD [28] and representative of a fAD-linked APP misprocessing ( Supplementary Fig. 2 ). The 6E10+4G8 SELDI-TOF MS method reveals in 7PA2 CM, the complex profile of Aβ monomeric peptides and of Aβ truncated forms but does not detect immunoproteomic peaks corresponding to AβOs. Thus, we investigated the patterns of soluble Aβ also by other approaches, such as western blot (WB) or DB. The WB analysis of straight (non-concentrated) 7PA2 CM shows that the Aβ oligomeric bands are a small fraction (<20%) of total soluble Aβ species, which mainly run in the gels as monomeric bands ( Supplementary Fig. 3 ). Accordingly, the biologically relevant LDS/SDS-stable Aβ dimers and trimers were previously recognized in 7PA2 CM as a small pool of total soluble Aβ species only upon immunoprecipitation enrichment [23] , [24] . Here, in a new way, we were able to detect LDS/SDS-stable Aβ dimers and trimers by a direct WB analysis of 7PA2 CM ( Supplementary Fig. 3 ), with a major sensitivity if the CM is previously subjected to concentration steps. We demonstrated that the dimeric and trimeric bands are Aβ-specific being selectively abolished by cell pretreatment with a γ-secretase inhibitor (L-685,458) [29] and being recognized by independent anti-Aβ antibodies (6E10 and 4G8) raised against different Aβ epitopes ( Supplementary Figs 4,5 ). Finally, we established a new AβO-specific DB assay, based on the use of scFvA13, and of the other conformation-sensitive anti-AβO scFvIm3 (ref. 13 ), as primary antibodies ( Supplementary Fig. 6 ). The scFv-based DB can selectively detect both extracellular and intracellular Aβ conformers ( Supplementary Figs 6,7 ). Of note, the DB approach is essential to analyse the intracellular pools of AβOs, hardly detectable by WB both for sensitivity limits and for the main cross-reactivity of the anti-Aβ 6E10 and 4G8 with a large number of intracellular APP fragments ( Supplementary Fig. 7a ). On the other hand, the anti-Aβ WB is a good method to detect Aβ monomeric bands, both in lysates and microsomes ( Supplementary Fig. 7b ), which are representative of the largest pool of intracellular Aβ species (both monomers and LDS/SDS unstable oligomers). Targeting the scFvA13 intrabody to the ER The scFvA13 intrabody was targeted to the early secretory pathway exploiting the ER retention/retrieval KDEL system. The subcellular localization of scFvA13-KDEL was confirmed by indirect immunofluorescence to be mainly in the ER and partially in the cis-Golgi ( Fig. 2a ). The effective enrichment in the ER was further demonstrated through the WB analysis of different subcellular vesicles derived by microsome fractionation of 7PA2 scFvA13-KDEL transfectants ( Fig. 2b ). Consistent with its retention in the ER, the scFvA13-KDEL was found not to be secreted in the extracellular medium ( Fig. 2c ). Of note, the scFvA13-KDEL intrabody does not perturb the expression levels of endogenous ER KDEL-bearing proteins or chaperones, and does not induce ER stress in 7PA2 and other cell lines (as measured by the unchanged levels of BiP) ( Fig. 2d ). 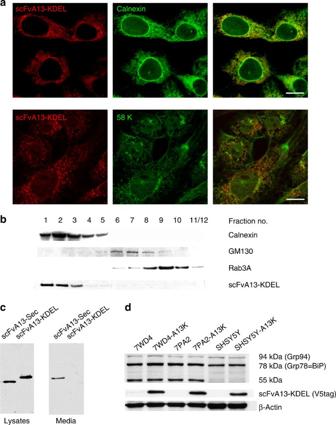Figure 2: The intrabody scFvA13-KDEL is targeted to the ER. (a) Confocal analysis of 7PA2 cells stably expressing the scFvA13-KDEL intrabody (7PA2-A13K cells). The intrabody was detected by indirect immunofluorescence through its C-terminal V5 tag by using an anti-V5 as a primary antibody (left panels). The middle panels show, from the top the ER marker calnexin and the Golgi marker protein 58K. The panels on the right show the respective merged images (scFvA13-KDEL with calnexin or 58K) with a major co-localization of scFvA13-KDEL intrabody with calnexin, and a partial co-localization of scFvA13-KDEL intrabody with 58K, indicating the preferential KDEL-mediated ER localization of the intrabody. Scale bar, 10 μm, magnification × 63. (b) WB analysis for calnexin (ER), GM130 (Golgi) and Rab3A (secretory vesicles) of a representative microsome fractionation of 7PA2-A13K cells. The scFvA13-KDEL intrabody is detected in the ER-enriched fractions. (c) WB analysis (blot with anti-V5) of lysates and of CM of representative 7PA2 clones stably expressing the scFvA13-KDEL or the scFvA13 secretory intrabody. The intrabody KDEL expressing cells do not secrete scFv protein in the culture media (no WB detection even in CM 15 × concentrated). (d) WB analysis (by using anti-KDEL as primary antibody) of KDEL proteins in 7WD4, 7PA2 and human neuroblastoma SHSY5Y, expressing or not the scFvA13-KDEL intrabody (steady-state levels). The expression of the intrabody KDEL does not perturb the expression of other KDEL proteins, such as the ER chaperones (that is, Grp78 or BiP and Grp94), showing it does not induce ER stress (BiP levels unchanged). WB of β-Actin and of scFv (by anti-V5) is also shown. Figure 2: The intrabody scFvA13-KDEL is targeted to the ER. ( a ) Confocal analysis of 7PA2 cells stably expressing the scFvA13-KDEL intrabody (7PA2-A13K cells). The intrabody was detected by indirect immunofluorescence through its C-terminal V5 tag by using an anti-V5 as a primary antibody (left panels). The middle panels show, from the top the ER marker calnexin and the Golgi marker protein 58K. The panels on the right show the respective merged images (scFvA13-KDEL with calnexin or 58K) with a major co-localization of scFvA13-KDEL intrabody with calnexin, and a partial co-localization of scFvA13-KDEL intrabody with 58K, indicating the preferential KDEL-mediated ER localization of the intrabody. Scale bar, 10 μm, magnification × 63. ( b ) WB analysis for calnexin (ER), GM130 (Golgi) and Rab3A (secretory vesicles) of a representative microsome fractionation of 7PA2-A13K cells. The scFvA13-KDEL intrabody is detected in the ER-enriched fractions. ( c ) WB analysis (blot with anti-V5) of lysates and of CM of representative 7PA2 clones stably expressing the scFvA13-KDEL or the scFvA13 secretory intrabody. The intrabody KDEL expressing cells do not secrete scFv protein in the culture media (no WB detection even in CM 15 × concentrated). ( d ) WB analysis (by using anti-KDEL as primary antibody) of KDEL proteins in 7WD4, 7PA2 and human neuroblastoma SHSY5Y, expressing or not the scFvA13-KDEL intrabody (steady-state levels). The expression of the intrabody KDEL does not perturb the expression of other KDEL proteins, such as the ER chaperones (that is, Grp78 or BiP and Grp94), showing it does not induce ER stress (BiP levels unchanged). WB of β-Actin and of scFv (by anti-V5) is also shown. Full size image The effect of scFvA13-KDEL on the extracellular pools of Aβ and AβOs To better study the effects of scFvA13-KDEL on the biochemistry of Aβ, AβOs and APP, we first established 7PA2 cells stably expressing the intrabody scFvA13-KDEL, referred to as 7PA2-A13K cells. The comparative WB analysis of straight CM from 7PA2 and 7PA2-A13K cells does not reveal significant differences in the levels of Aβ monomeric bands, which are representative of the largest amount of soluble Aβ species (monomers and LDS/SDS unstable oligomers) ( Supplementary Fig. 3 ). Instead, the amount of LDS/SDS-stable Aβ dimers and trimers secreted from 7PA2 cells (detected in concentrated CM) is significantly reduced (~\n60% in 4G8-WB and ~\n70% in 6E10-WB) by the expression of the scFvA13-KDEL intrabody ( Fig. 3a ; Supplementary Fig. 5 ). Similarly, the secreted oligomeric conformers, measured by scFv-DB assay in CM, are significantly reduced (70–80%) in 7PA2-A13K ( Fig. 3b ; Supplementary Fig. 6 ). Of note, the similar ratio of AβOs decrease, measured by WB (selective for Aβ dimers and trimers with respect to the monomeric Aβ bands) and by DB, further attests the oligomeric specificity of the scFv-based DB assay (in addition to the experimental control of γ-secretase inhibitor treatment, Supplementary Fig. 6 ). 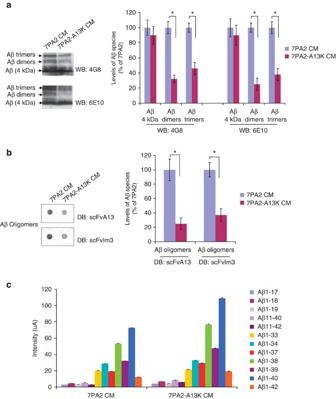Figure 3: Impact of scFvA13-KDEL in 7PA2 cells on the extracellular patterns of Aβ species. (a) WB analysis of secreted AβOs in the CM of 7PA2 cells and of 7PA2 stably expressing the scFvA13-KDEL intrabody (7PA2-A13K). LDS/SDS-stable Aβ dimers and Aβ trimers were detected by WB using two different anti-Aβ mAbs, mAb 4G8 (against a.a. 17–25 of Aβ) and mAb 6E10 (against a.a. 3–9 of Aβ), as primary antibodies (see alsoSupplementary Fig. 5). Aβ dimers and Aβ trimers are significantly reduced in 7PA2-A13K, whereas no significant changes in the 4 kDa Aβ bands (deriving both from monomers and LDS/SDS unstable oligomers) are observed (see alsoSupplementary Figs. 3,5). The histogram shows the levels of Aβ species in 7PA2-A13K CM in comparison with 7PA2 CM (at 100) obtained from densitometric values of bands and normalized as discussed in the method section and in theSupplementary Fig. 5. Mean values±s.e.m.,n=4, *P<0.01, Student’st-test. (b) DB analysis of AβOs in CM were done by using the conformation-sensitive and sequence-specific scFvA13 or scFvIm3 anti-AβOs13as primary antibodies (and detected through anti-His tag). The levels of AβOs are significantly decreased in 7PA2-A13K CM, in comparison with 7PA2 CM, similarly to those of Aβ dimers and Aβ trimers (measured by WB). The histogram shows the levels of AβOs in 7PA2-A13K CM in comparison with 7PA2 CM (at 100) obtained from densitometric values of dots and normalized as discussed in the method section. Mean values±s.e.m.,n=4, *P<0.01, Student’st-test. (c) Immunoproteomic analysis of secreted Aβ monomers and fragments. The levels of N- and C-terminally truncated Aβ monomers, measured by 6E10+4G8 SELDI-TOF MS, are significantly increased in 7PA2-A13K CM, in comparison with 7PA2 CM (all ratios inSupplementary Table 2). The most abundant Aβ species are increased by 53.1±1.6% (Aβ1-37), 44.2±1.1% (Aβ1-38), 48.6±0.9% (Aβ1-39), 50±0.3% (Aβ1-40), 59±3.3% (Aβ1-42), respectively. The histogram shows the intensity (microampere, uA) of single proteomic peaks. Mean values±s.e.m.,n=4,P<0.001, Student’st-test. Figure 3: Impact of scFvA13-KDEL in 7PA2 cells on the extracellular patterns of Aβ species. ( a ) WB analysis of secreted AβOs in the CM of 7PA2 cells and of 7PA2 stably expressing the scFvA13-KDEL intrabody (7PA2-A13K). LDS/SDS-stable Aβ dimers and Aβ trimers were detected by WB using two different anti-Aβ mAbs, mAb 4G8 (against a.a. 17–25 of Aβ) and mAb 6E10 (against a.a. 3–9 of Aβ), as primary antibodies (see also Supplementary Fig. 5 ). Aβ dimers and Aβ trimers are significantly reduced in 7PA2-A13K, whereas no significant changes in the 4 kDa Aβ bands (deriving both from monomers and LDS/SDS unstable oligomers) are observed (see also Supplementary Figs. 3,5 ). The histogram shows the levels of Aβ species in 7PA2-A13K CM in comparison with 7PA2 CM (at 100) obtained from densitometric values of bands and normalized as discussed in the method section and in the Supplementary Fig. 5 . Mean values±s.e.m., n =4, * P <0.01, Student’s t -test. ( b ) DB analysis of AβOs in CM were done by using the conformation-sensitive and sequence-specific scFvA13 or scFvIm3 anti-AβOs [13] as primary antibodies (and detected through anti-His tag). The levels of AβOs are significantly decreased in 7PA2-A13K CM, in comparison with 7PA2 CM, similarly to those of Aβ dimers and Aβ trimers (measured by WB). The histogram shows the levels of AβOs in 7PA2-A13K CM in comparison with 7PA2 CM (at 100) obtained from densitometric values of dots and normalized as discussed in the method section. Mean values±s.e.m., n =4, * P <0.01, Student’s t -test. ( c ) Immunoproteomic analysis of secreted Aβ monomers and fragments. The levels of N- and C-terminally truncated Aβ monomers, measured by 6E10+4G8 SELDI-TOF MS, are significantly increased in 7PA2-A13K CM, in comparison with 7PA2 CM (all ratios in Supplementary Table 2 ). The most abundant Aβ species are increased by 53.1±1.6% (Aβ1-37), 44.2±1.1% (Aβ1-38), 48.6±0.9% (Aβ1-39), 50±0.3% (Aβ1-40), 59±3.3% (Aβ1-42), respectively. The histogram shows the intensity (microampere, uA) of single proteomic peaks. Mean values±s.e.m., n =4, P <0.001, Student’s t -test. Full size image In contrast to the reduction of AβOs measured in the CM of 7PA2-A13K cells, the immunoproteomic analysis of 7PA2-A13K CM (by 6E10+4G8 SELDI-TOF MS) shows a significant increase of Aβ monomeric species, with respect to 7PA2 CM ( Fig. 3c ). Relevantly, the expression of scFvA13-KDEL does not alter the profile of γ-secretase-generated Aβ products (species of 37–42 amino-acid length) in 7PA2 cells, but leads, instead, to a similar increase in the absolute amounts of all Aβ species ( Fig. 3c , Supplementary Table 2 ). Thus, the intracellular expression of scFvA13-KDEL determines a selective and significant reduction of extracellular AβOs accompanied by an opposite increase of secreted Aβ monomers and truncated forms. While it is difficult to establish a precise quantitative balance between these two independent Aβ pools, our results show that their variations are likely mutually complementary. Modulation of the intracellular Aβ and AβOs pools by the scFvA13-KDEL We evaluated the effects of the scFvA13-KDEL expression on the intracellular pools of Aβ and AβOs by WB and DB analyses. The anti-Aβ WB analysis allows concluding that the intracellular Aβ monomeric bands are not significantly changed in 7PA2-A13K lysates ( Fig. 4 ), neither in total microsomes ( Supplementary Fig. 7b ), while the levels of intracellular AβO conformers (selectively detected by DB analysis in cell lysates) are significantly decreased ( Fig. 4 , Supplementary Fig. 7b ). Of note, also the intracellular oligomers detected (in DB) by the independent A11 polyclonal antibody [21] , known to recognize the so-called ‘prefibrillar oligomers’ (larger than dimers and trimers) [30] , are found to be decreased in 7PA2-A13K cells ( Fig. 4 ). 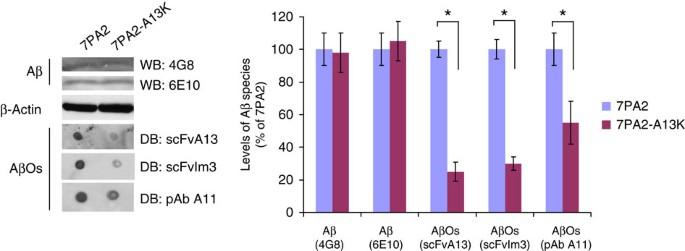Figure 4: The intracellular Aβ and AβOs in 7PA2-A13K cells. WB analysis of Aβ (blot with 6E10 and 4G8) and DB analysis of AβOs (blot with the anti-AβOs scFvA13 and scFvIm3 and with the generic anti-oligomers pAbA11) in 7PA2 and 7PA2-A13K cell lysates. In WB, the Aβ monomeric bands do not show significant changes (nor in total microsomes, seeSupplementary Fig. 7b). The intracellular AβOs, measured by scFvA13 or scFvIm3 or pAbA11 DB on cell lysates, show significantly decreased levels in 7PA2-A13K cells in comparison with 7PA2 cells. The histogram shows the Aβ and AβO levels in 7PA2-A13K lysates in comparison with 7PA2 cells (at 100) obtained from densitometric values of bands and dots and normalized versus β-Actin and versus the amount of total proteins in lysates. Mean values±s.e.m.,n=3, *P<0.01, Student’st-test. Figure 4: The intracellular Aβ and AβOs in 7PA2-A13K cells. WB analysis of Aβ (blot with 6E10 and 4G8) and DB analysis of AβOs (blot with the anti-AβOs scFvA13 and scFvIm3 and with the generic anti-oligomers pAbA11) in 7PA2 and 7PA2-A13K cell lysates. In WB, the Aβ monomeric bands do not show significant changes (nor in total microsomes, see Supplementary Fig. 7b ). The intracellular AβOs, measured by scFvA13 or scFvIm3 or pAbA11 DB on cell lysates, show significantly decreased levels in 7PA2-A13K cells in comparison with 7PA2 cells. The histogram shows the Aβ and AβO levels in 7PA2-A13K lysates in comparison with 7PA2 cells (at 100) obtained from densitometric values of bands and dots and normalized versus β-Actin and versus the amount of total proteins in lysates. Mean values±s.e.m., n =3, * P <0.01, Student’s t -test. Full size image Thus, the reduction of secreted AβOs determined by the expression of scFvA13-KDEL occurs without a concomitant intracellular accumulation of Aβ and with a reduction of intracellular AβO conformers, detected by scFvA13, scFvIm3 and A11 likely as distinct pools of AβOs. Results can be explained by an interference of the scFvA13-KDEL intrabody in the formation of stable AβOs in the ER, highlighting the relevance of intracellular (as opposed to the extracellular) Aβ oligomerization process in the overall balance of AβOs. We conclude that the ER-assembled AβOs are a consistent source of those secreted extracellularly and of those found intracellularly. Of note, the expression of an Aβ-unrelated intrabody (scFvR4-KDEL used as negative control) in 7PA2 cells, has no effect on the levels of extra- and intracellular Aβ or AβOs ( Supplementary Fig. 8 ). ScFvA13-KDEL intrabody does not affect the APP metabolism To further characterize the cellular mechanisms leading to the observed changes in Aβ/AβOs levels in the 7PA2-A13K cells (summarized in the Supplementary Table 3 ), we investigated whether the intrabody has a direct or indirect interference on the expression, maturation and processing of APP, processes which tightly influence the levels of secreted Aβ ( Fig. 5 ). 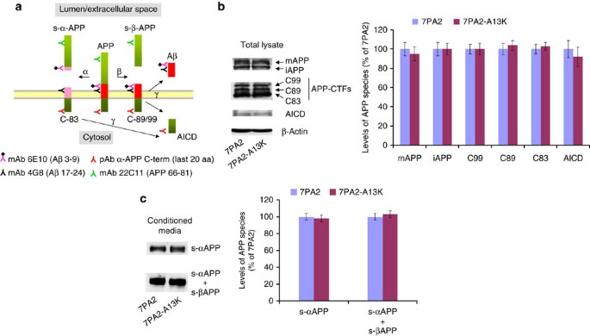Figure 5: Effects of the intrabody on the expression, maturation and processing of APP. (a) Scheme of APP fragments generated during APP–RIP and epitopes recognized by different anti-Aβ/APP antibodies used. (b) WB (anti-APP C-terminal) for full-length APP and for APP–CTFs in 7PA2 and in 7PA2-A13K lysates. i-APP and m-APP indicate the immature (N-glycosylated) and mature (N+O-glycosylated) forms of APP. The APP–CTFs are: C83, deriving from α-, C89 and C99 from β-secretase cleavage. The AICD derives from γ-secretase activities (seea). The histogram shows the levels of different APP forms in 7PA2-A13K lysates in comparison with 7PA2 cells (at 100) obtained from densitometric values of bands and normalized versus β-Actin. Mean values±s.e.m.,n=3. No significant differences between 7PA2 and 7PA2-A13K cells were observed. (c) WB for soluble sα-APP (mAb 6E10) and sα-APP+sβ-APP (anti-APP N-terminal mAb 22C11) in 7PA2 and in 7PA2-A13K CM, deriving from α- and β- secretase APP-cleavage. The histogram shows the levels of soluble APPs in 7PA2-A13K CM in comparison with 7PA2 CM (at 100) obtained from densitometric values of bands and normalized as discussed in the method section and in theSupplementary Fig. 5. Mean values±s.e.m.,n=3. No significant changes of soluble APPs were observed in 7PA2-A13K cells in comparison with 7PA2 cells. Figure 5: Effects of the intrabody on the expression, maturation and processing of APP. ( a ) Scheme of APP fragments generated during APP–RIP and epitopes recognized by different anti-Aβ/APP antibodies used. ( b ) WB (anti-APP C-terminal) for full-length APP and for APP–CTFs in 7PA2 and in 7PA2-A13K lysates. i-APP and m-APP indicate the immature (N-glycosylated) and mature (N+O-glycosylated) forms of APP. The APP–CTFs are: C83, deriving from α-, C89 and C99 from β-secretase cleavage. The AICD derives from γ-secretase activities (see a ). The histogram shows the levels of different APP forms in 7PA2-A13K lysates in comparison with 7PA2 cells (at 100) obtained from densitometric values of bands and normalized versus β-Actin. Mean values±s.e.m., n =3. No significant differences between 7PA2 and 7PA2-A13K cells were observed. ( c ) WB for soluble sα-APP (mAb 6E10) and sα-APP+sβ-APP (anti-APP N-terminal mAb 22C11) in 7PA2 and in 7PA2-A13K CM, deriving from α- and β- secretase APP-cleavage. The histogram shows the levels of soluble APPs in 7PA2-A13K CM in comparison with 7PA2 CM (at 100) obtained from densitometric values of bands and normalized as discussed in the method section and in the Supplementary Fig. 5 . Mean values±s.e.m., n =3. No significant changes of soluble APPs were observed in 7PA2-A13K cells in comparison with 7PA2 cells. Full size image The steady-state levels of full-length APP and of APP C-terminal fragments (CTFs) in total lysates ( Fig. 5b ), as well as of soluble α-APP and β-APP in the extracellular medium ( Fig. 5c ), are similar in 7PA2 and in 7PA2-A13K cells. Likewise, in comparative subcellular fractionation studies, the scFvA13-KDEL intrabody does not affect the intracellular maturation and processing of APP, assessed by evaluating the compartment-specific (ER versus Golgi) N- and O-glycosylation of APP and the CTFs levels ( Fig. 6a ). Finally, the subcellular activities of α- β- and γ-secretase were found not to be affected by the scFvA13-KDEL intrabody, as measured in comparative analyses of 7PA2 and 7PA2-A13K cells ( Fig. 6b,c ). In detail, the γ-secretase activity was assayed in subcellular ER-enriched fractions after their incubation for 2 h at 37 °C, by measuring the selective reduction of the APP–CTFs and the appearance of the APP intracellular domain (AICD) ( Fig. 6b ) (as previously described [31] ). Furthermore, we established an assay to determine both γ-secretase and α-, β-secretases activities through a reversible block of intracellular trafficking from ER to Golgi with Brefeldin A (BFA). One or four hours of treatment with BFA determines: (i) a time-dependent reduction of APP–CTFs (almost complete after 4 h of treatment) indicative of γ-secretase processing; (ii) a significant change in the ratio of immature/mature APP forms, with a prevalence of the immature one, indicative of the block of APP in the ER. After a 2 h washout of BFA: (i) the APP–CTFs are reestablished or de novo generated (indicative of α-, β-secretases activities likely in post-ER compartments); (ii) the maturation (glycosylation) of full-length APP, previously prevented by the BFA treatment, is restored ( Fig. 6c ). 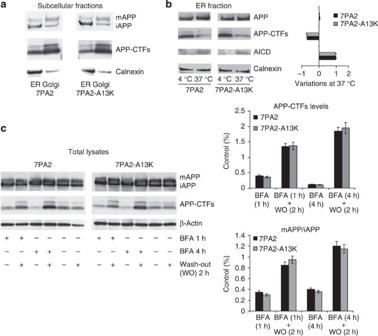Figure 6: The scFvA13-KDEL does not alter the subcellular maturation and processing of APP. (a) WB analysis (anti-APP C-terminal) of the compartment-specific APP maturation and processing in representative subcellular fractions (ER or Golgi enriched) of 7PA2 and 7PA2-A13K cells. The ER and Golgi specificities (such as the different ratio i-APP/m-APP, and the different CTFs levels) are similar in 7PA2 and 7PA2-A13K cells. (b) γ-secretase activity in subcellular ER-enriched fractions of 7PA2 and 7PA2-A13K cells assayed by WB (anti-APP C-terminal). Freshly prepared ER-enriched fractions are incubated for 2 h at 37 °C or at 4 °C, to allow (37 °C) or not (4 °C) specific γ-secretases APP cleavages at the γ- andε-sites, respectively measured by the selective reduction of the APP–CTFs C99-C83 (but not of the full-length APP) and by the appearance of the AICD. The histogram shows the variations at 37 °C of APP, APP–CTFs and AICD (densitometric values of WB bands normalized versus calnexin). Mean values±s.e.m.,n=3. No significant differences between 7PA2 and 7PA2-A13K cells were observed. (c) Total cell lysates WB analysis of APP and APP–CTFs (anti-APP C-terminal), in experiments of reversible block of intracellular trafficking from ER to Golgi complex: transient (1 or 4 h) BFA treatment induces a reduction of APP–CTFs, which can be completely reversed after a 2 h BFA washout. The reduction of APP–CTFs is indicative of γ-secretase processing, whereas the re-establishment (orde novogeneration) of CTFs levels is indicative of α-, β-secretases activities. The upper histogram shows the variations at of APP–CTFs (densitometric values of WB bands normalized versus β-Actin, and represented as % of corresponding control). Mean values±s.e.m.,n=3. No significant differences between 7PA2 and 7PA2-A13K cells were observed. In addition, as expected, 1 or 4 h BFA treatment blocks also the maturation of the full-length APP. The lower histogram shows the variations of the ratios m-APP/iAPP (calculated from densitometric values of WB bands normalized versus β-Actin, and represented as % of corresponding control). Mean values±s.e.m.,n=3. No significant differences between 7PA2 and 7PA2-A13K cells were observed. Figure 6: The scFvA13-KDEL does not alter the subcellular maturation and processing of APP. ( a ) WB analysis (anti-APP C-terminal) of the compartment-specific APP maturation and processing in representative subcellular fractions (ER or Golgi enriched) of 7PA2 and 7PA2-A13K cells. The ER and Golgi specificities (such as the different ratio i-APP/m-APP, and the different CTFs levels) are similar in 7PA2 and 7PA2-A13K cells. ( b ) γ-secretase activity in subcellular ER-enriched fractions of 7PA2 and 7PA2-A13K cells assayed by WB (anti-APP C-terminal). Freshly prepared ER-enriched fractions are incubated for 2 h at 37 °C or at 4 °C, to allow (37 °C) or not (4 °C) specific γ-secretases APP cleavages at the γ- and ε -sites, respectively measured by the selective reduction of the APP–CTFs C99-C83 (but not of the full-length APP) and by the appearance of the AICD. The histogram shows the variations at 37 °C of APP, APP–CTFs and AICD (densitometric values of WB bands normalized versus calnexin). Mean values±s.e.m., n =3. No significant differences between 7PA2 and 7PA2-A13K cells were observed. ( c ) Total cell lysates WB analysis of APP and APP–CTFs (anti-APP C-terminal), in experiments of reversible block of intracellular trafficking from ER to Golgi complex: transient (1 or 4 h) BFA treatment induces a reduction of APP–CTFs, which can be completely reversed after a 2 h BFA washout. The reduction of APP–CTFs is indicative of γ-secretase processing, whereas the re-establishment (or de novo generation) of CTFs levels is indicative of α-, β-secretases activities. The upper histogram shows the variations at of APP–CTFs (densitometric values of WB bands normalized versus β-Actin, and represented as % of corresponding control). Mean values±s.e.m., n =3. No significant differences between 7PA2 and 7PA2-A13K cells were observed. In addition, as expected, 1 or 4 h BFA treatment blocks also the maturation of the full-length APP. The lower histogram shows the variations of the ratios m-APP/iAPP (calculated from densitometric values of WB bands normalized versus β-Actin, and represented as % of corresponding control). Mean values±s.e.m., n =3. No significant differences between 7PA2 and 7PA2-A13K cells were observed. Full size image All these assays show that in 7PA2 cells, the anti-AβOs scFvA13-KDEL does not affect the maturation and processing of APP, not even during its trafficking in the early secretory pathway where the intrabody resides, shuttling between ER and cis-Golgi. Remarkably, also in other cell lines (7WD4 and SHSY5Y) with lower or negligible levels of AβOs, scFvA13-KDEL does not interfere with the physiological APP processing ( Supplementary Fig. 9 ). In conclusion, our data demonstrate that the scFvA13-KDEL intrabody acts effectively and selectively on the levels of extra- and intracellular pools of AβOs, with no interference with APP expression, maturation or processing. This molecular and subcellular selectivity represents a significant experimental advance to modulate the levels of Aβ peptides, in comparison with widely used approaches of γ-secretase inhibition. Indeed, as expected, we found that in 7PA2 cells the γ-secretase inhibitor L-685,458 (ref. 29 ) dramatically decreases the production of Aβ and, consequently, of AβOs, but massively increases the levels of α- and β-CTFs, altering also their subcellular distribution, and the levels of soluble APPs ( Supplementary Fig. 10 ). The lack of interference of the intrabody on the APP cellular biochemistry is noteworthy due to several functions of APP-derived fragments (that is, of soluble APPs and of AICD) [32] . ScFvA13-KDEL selectively binds AβOs in the ER In order to explore the selective mechanism of AβO modulation, we first investigated the interaction of the intrabody with subcellularly localized Aβ/AβOs species, by microsome fractionation of 7PA2-A13K cells, followed by co-immunoprecipitation (co-IP) and WB analyses. We demonstrated the intrabody-mediated selective pulldown of LDS/SDS-stable Aβ dimers, trimers and small oligomers (<20 kDa), but not of Aβ monomers, neither of the full-length APP, in the ER-enriched fractions of 7PA2-A13K cells ( Fig. 7a ). The AβO pulldown was successful when freshly prepared microsome vesicles were subjected to a preliminary step of chemical cross-linking; this suggests a transient nature of the AβO-intrabody complexes (consistent with a chaperone-like interaction of the intrabody). 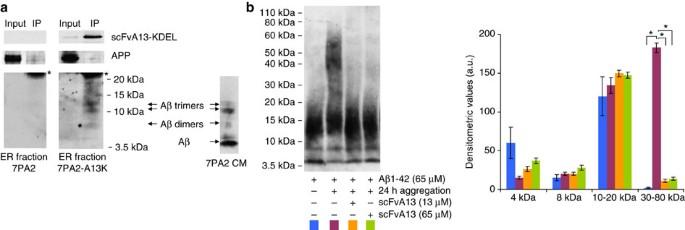Figure 7: Intrabody binding of AβOs in the ER and interference of scFvA13 with Aβ assemblyin vitro. (a) Intrabody-mediated selective pulldown of AβOs: co-IP of scFvA13-KDEL intrabody with Aβ dimers, Aβ trimers and larger AβOs (<20 kDa) but not with Aβ monomers nor APP, from an ER-enriched fraction of 7PA2-A13K cells (7PA2 cells as intrabody negative control). The co-IP was obtained by an anti-V5 coupled resin, to bind the C-terminal V5 tag of the intrabody and blotted to detect the different Aβ species and APP (mAb 6E10) and for the intrabody (anti-V5). * indicates the light chain of the anti-V5 IP antibody. On the right, representative Aβ bands detected (by 6E10-WB) in 7PA2 CM in the 3.5–15 kDa range. (b) WB analysis (rabbit mAb anti-Aβ) of Aβ assembledin vitrowith or without scFvA13. The human Aβ1-42 peptide (65 μM) was aggregated at 22 °C for 24 h without scFvA13, or in the presence of substoichiometric (13 μM, ratio Aβ:scFv, 1:5) or stoichiometric concentrations (65 μM) of scFvA13. According to previous reports47, after thein vitroassembly, synthetic Aβ1-42 shows a pattern of HMW oligomers (30–80 kDa) absent at the early steps of aggregation (in which Aβ monomers and LMW oligomers (<20 kDa) prevail). Of note, the co-presence of LMW oligomers and monomers cannot be ruled out in starting solutions of synthetic Aβ70, being these species in rapid equilibrium and determining variability on the levels of Aβ monomers measured. Both sub- and stoichiometric concentrations of scFvA13 during the assembly of Aβ1-42 determine the following: (i) the lack of formation of HMW AβOs; (ii) a pattern of LMW AβOs similar to that at the early steps of aggregation. This shows that the scFvA13 interferes with critical conformational changes during the early assembly, avoiding the formation of larger AβOs. The histogram shows the variations of Aβ species obtained from densitometric analysis. Mean values±s.e.m.,n=3; *P<0.01 (Student’st-test). Figure 7: Intrabody binding of AβOs in the ER and interference of scFvA13 with Aβ assembly in vitro . ( a ) Intrabody-mediated selective pulldown of AβOs: co-IP of scFvA13-KDEL intrabody with Aβ dimers, Aβ trimers and larger AβOs (<20 kDa) but not with Aβ monomers nor APP, from an ER-enriched fraction of 7PA2-A13K cells (7PA2 cells as intrabody negative control). The co-IP was obtained by an anti-V5 coupled resin, to bind the C-terminal V5 tag of the intrabody and blotted to detect the different Aβ species and APP (mAb 6E10) and for the intrabody (anti-V5). * indicates the light chain of the anti-V5 IP antibody. On the right, representative Aβ bands detected (by 6E10-WB) in 7PA2 CM in the 3.5–15 kDa range. ( b ) WB analysis (rabbit mAb anti-Aβ) of Aβ assembled in vitro with or without scFvA13. The human Aβ1-42 peptide (65 μM) was aggregated at 22 °C for 24 h without scFvA13, or in the presence of substoichiometric (13 μM, ratio Aβ:scFv, 1:5) or stoichiometric concentrations (65 μM) of scFvA13. According to previous reports [47] , after the in vitro assembly, synthetic Aβ1-42 shows a pattern of HMW oligomers (30–80 kDa) absent at the early steps of aggregation (in which Aβ monomers and LMW oligomers (<20 kDa) prevail). Of note, the co-presence of LMW oligomers and monomers cannot be ruled out in starting solutions of synthetic Aβ [70] , being these species in rapid equilibrium and determining variability on the levels of Aβ monomers measured. Both sub- and stoichiometric concentrations of scFvA13 during the assembly of Aβ1-42 determine the following: (i) the lack of formation of HMW AβOs; (ii) a pattern of LMW AβOs similar to that at the early steps of aggregation. This shows that the scFvA13 interferes with critical conformational changes during the early assembly, avoiding the formation of larger AβOs. The histogram shows the variations of Aβ species obtained from densitometric analysis. Mean values±s.e.m., n =3; * P <0.01 (Student’s t -test). Full size image The binding selectivity of scFvA13-KDEL intrabody for AβOs in living cells, with respect to the monomeric Aβ, is in accordance with the in vitro oligomer-selective discrimination and conformation binding properties of the scFvA13 (ref. 13 ), but the fact that we could prove it in the intracellular environment is noteworthy. Furthermore, the binding selectivity with respect to the APP further suggests that, in the ER lumen, the Aβ moiety in the context of APP is not recognized by the scFvA13-KDEL intrabody, in line with the lack of interference with APP processing and maturation ( Figs 5 , 6 ). We suggest that the primary action of scFvA13-KDEL intrabody is to bind to early-assembled, possibly transient, AβO conformers (here detected in the co-IP/WB analysis as SDS/LDS-stable Aβ dimers and trimers and small AβOs), but not to the free Aβ monomers. This could inhibit a further Aβ oligomerization, most likely due to the interference with critical seeding defined by the bound AβO conformers. The significant reduction of intracellular pool of AβOs measured by A11 antibody (see Fig. 4 ), which preferentially recognizes prefibrillar AβOs larger than dimers and trimers [30] , is also in accordance with this proposed mechanism. The co-IP results ( Fig. 7a ) and the DB immunoreactivity of cell lysates with A11, scFvA13 and scFvIm3 ( Fig. 4 ) (the latter confirmed as Aβ-specific by the γ-secretase inhibitor treatment ( Supplementary Fig. 7b )), demonstrate that AβOs larger than dimers and trimers exist in the intracellular environment of 7PA2 cells. We conclude that the intrabody-mediated interference in the ER with the dynamic pool of intracellular AβOs, including oligomers larger than Aβ dimers and trimers, can influence also the balance of extracellular AβOs, which are mainly detected as LDS/SDS-stable dimers and trimers. The scFvA13 interferes with AβOs assembly in vitro We studied next the effects of scFvA13 (used as purified protein) on the formation of AβOs or on preformed AβOs in vitro . Indeed, while considering obvious and well-known differences between natural and synthetic Aβ samples (that is, the high concentration of synthetic Aβ used in vitro and the different appearance of Aβ assemblies) [33] such in vitro study could help interpreting the mechanism of conformational interference of scFvA13-KDEL intrabody. We demonstrated that the scFvA13, both at stoichiometric and substoichiometric ratios with the Aβ1-42 monomeric peptide, strongly inhibits the assembly of AβOs in vitro . Indeed, in the presence of scFvA13, we observed the lack of formation of high-molecular weight (HMW) AβOs (30–80 kDa in WB analysis) from a starting solution where Aβ monomers and low-molecular weight (LMW) oligomers (<20 kDa) are in rapid equilibrium ( Fig. 7b ). Thus, the scFvA13 blocks the assembly from LMW towards HMW AβOs ( Fig. 7b ). In addition, we studied whether and how the scFvA13 acts on preformed AβOs. When incubated with scFvA13, LMW and HMW AβOs undergo a change of their assembly state, as revealed by the reduction of their MWs with a concomitant significant increase of free Aβ monomers (in a scFv concentration-dependent manner) ( Supplementary Fig. 11 ). Both these in vitro observations (dynamic interference in assembly and disassembly pathways) support our hypothesis on the mechanism of action of the scFvA13-KDEL intrabody on AβO conformers and are in accordance with the binding and pulldown into the ER and with measured overall modulation of Aβ/AβOs levels in cells (reduction of AβOs and the increase of secreted Aβ monomers). Intracellular fate of scFvA13-KDEL In order to support the mechanism by which the scFvA13-KDEL intrabody intercepts early AβO conformers in the ER and acts as a conformational-sensitive and chaperon-like assembly modulator, we better characterized the subcellular localization of scFvA13-KDEL and its possible delivery to pathways of cellular degradation. We found that the intrabody does not localize in trans-Golgi network (TGN), neither in early nor late endosomes and in lysosomes (as demonstrated by indirect immunofluorescence, by the lack of co-localization with the subcellular markers TGN46, Rab5, Rab7 or LAMP-1, respectively) ( Fig. 8a ). Thus, the intrabody, as expected for a physiological and non-altered KDEL system, is mainly restricted into the ER excluding its localization in other endocytic vesicles which are crucially involved in recycling or degradation pathways. Of note, the TGN was recently identified as a crucial compartment for the synthesis of Aβ40 mainly due to the APP re-routing from the plasma membrane via the retromeric pathway [34] . Also endosomal, lysosomal and the secretory pathway (ER, Golgi) were demonstrated to be sites of Aβ production [7] . However, the precise localization of the scFvA13-KDEL in the ER (and, only partially, with cis-Golgi), as demonstrated, strongly support the view of a more confined action of the intrabody in these compartments. This formally establishes the ER (and cis-Golgi) as a major organelle where the control of Aβ oligomerization is crucial. 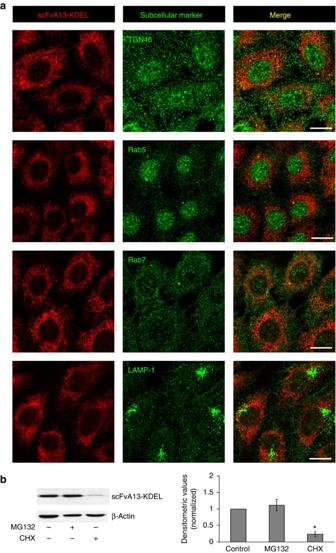Figure 8: The subcellular fate of scFvA13-KDEL intrabody. (a) Confocal analysis of 7PA2-A13K cells. The localization of scFvA13-KDEL (detected by using an anti-V5, seeFig. 2a) is showed in the left panels. The middle panels show the localization of different subcellular markers, from the top TGN46 (for the trans-Golgi network), Rab5 (for early endosomes), Rab7 (for late endosomes) and LAMP-1 (for lysosomes). The panels on the right show the respective merged images. Scale bar, 10 μm, magnification × 63. No significant co-localization of the ER-resident intrabody with any subcellular marker was observed, excluding mechanisms of mis- or re-localization of scFvA13-KDEL from the ER, or its sorting in recycling (endosomes-TGN) or degradation (lysosomes) pathways. (b) WB analysis (anti-V5 tag) of scFvA13-KDEL in 7PA2-A13K cells after 6 h MG132 (20 μM) treatment (to block the proteasome and study the ERAD pathway) or after 6 h cycloheximide (CHX) (40 μM) to block the protein synthesis. The histogram shows the levels of scFvA13-KDEL in the different treatments (values normalized from densitometric analysis of bands by ScionImage software). No significant changes in MG132 treatment were observed, excluding ERAD mechanisms. Comparative experiments show that a different version of the intrabody, referred to as scFvA13-degradin, undergoes significant ERAD (Supplementary Fig. 12). Mean values±s.e.m.,n=3; *P<0.01 (Student’st-test) in CHX treatment both versus control and versus MG132 treatment. Figure 8: The subcellular fate of scFvA13-KDEL intrabody. ( a ) Confocal analysis of 7PA2-A13K cells. The localization of scFvA13-KDEL (detected by using an anti-V5, see Fig. 2a ) is showed in the left panels. The middle panels show the localization of different subcellular markers, from the top TGN46 (for the trans-Golgi network), Rab5 (for early endosomes), Rab7 (for late endosomes) and LAMP-1 (for lysosomes). The panels on the right show the respective merged images. Scale bar, 10 μm, magnification × 63. No significant co-localization of the ER-resident intrabody with any subcellular marker was observed, excluding mechanisms of mis- or re-localization of scFvA13-KDEL from the ER, or its sorting in recycling (endosomes-TGN) or degradation (lysosomes) pathways. ( b ) WB analysis (anti-V5 tag) of scFvA13-KDEL in 7PA2-A13K cells after 6 h MG132 (20 μM) treatment (to block the proteasome and study the ERAD pathway) or after 6 h cycloheximide (CHX) (40 μM) to block the protein synthesis. The histogram shows the levels of scFvA13-KDEL in the different treatments (values normalized from densitometric analysis of bands by ScionImage software). No significant changes in MG132 treatment were observed, excluding ERAD mechanisms. Comparative experiments show that a different version of the intrabody, referred to as scFvA13-degradin, undergoes significant ERAD ( Supplementary Fig. 12 ). Mean values±s.e.m., n =3; * P <0.01 (Student’s t -test) in CHX treatment both versus control and versus MG132 treatment. Full size image We next investigated if the scFvA13-KDEL intrabody undergoes possible mechanisms of ER-associated degradation (ERAD) that acts through the ER to cytosol retrotranslocation of ER-resident proteins and their degradation by targeting the proteasome [35] . In principle, the ER-localized intrabody might escort the bound AβOs to the ERAD pathway. We observed, however, that in 7PA2-A13K cells, the levels of the intrabody do not change after 6-h treatment with the proteasome inhibitor MG132 (20 μM) ( Fig. 8b ). On the other hand, in 7PA2 cells stably expressing a different version of the intrabody, referred to as ‘scFvA13-degradin’ (specifically targeted to the ERAD system via C-terminal fusion with the moiety of SEL1L protein involved in the retrotranslocation process) [36] , we observed a significant increase of the intrabody levels after 6 h MG132 treatment ( Supplementary Fig. 12 ). Thus, the scFvA13-degradin undergoes ERAD and proteasome degradation, while the scFvA13-KDEL does not. As control, a 6-h treatment with cycloheximide (blocking the protein synthesis) dramatically reduces the levels of both scFvA13-KDEL ( Fig. 8b ) and scFvA13-degradin ( Supplementary Fig. 12 ) suggesting for both intrabody forms a short yet similar half-life. The short half-life of the intrabody scFvA13-KDEL is also confirmed by an in vitro assay on ER-enriched subcellular fractions, where the intrabody undergoes an almost complete degradation after 6 h of incubation at 37 °C ( Supplementary Fig. 13 ). The overall data suggest that the scFvA13-KDEL is mainly located in the ER, does not alter the APP maturation and processing, and does not undergo ERAD process. Furthermore, the short half-life of scFvA13-KDEL, together with its moderate levels of expression, prevents its accumulation in the ER and a consequent ER stress. We conclude that observed variations of AβO levels and the overall balance of secreted Aβ species are representative of a fine mechanism of conformational assembly modulation of AβO, which occurs in the ER (and in KDEL recycling compartments) where the intrabody intercepts critical conformers changing their oligomerizing fate, rather than their targeted degradation to proteasome or their subcellular re-targeting in other active endocytic pathways. Functional consequences of the intrabody interference with AβOs In order to investigate the functional consequences of the selective interference of the scFvA13-KDEL intrabody with specific pools of AβO conformers, we exploited two established experimental readouts on 7PA2 cells. The AβOs secreted by 7PA2 cells induce specific AD-related synaptic dysfunctions, when administered to primary neurons, brain slices or rodent brains [3] , [8] , [9] , [24] , [25] , [26] . In detail, in the primary hippocampal neurons, AβOs (contained in 7PA2 CM) can induce an impairment of the signalling mediated by extrasynaptic NR2B-containing NMDA receptors, modulating the ERK1/2 and CREB phosphorylation status [26] . Here, we demonstrate, in this experimental paradigm, that both ERK1/2 and CREB are largely dephosphorylated in the hippocampal neurons treated with 7PA2 CM but significantly less in those treated with 7PA2-A13K CM ( Fig. 9a ). This provides a functional demonstration that the AβO conformers targeted by the scFvA13-KDEL (and selectively immunodepleted in the 7PA2-A13K CM) are involved in the activation of a NR2B-NMDA extrasynaptic signalling, which is implicated in neurodegenerative cascades [37] . 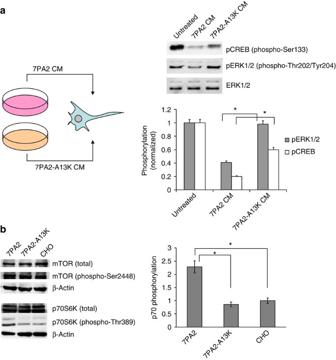Figure 9: Functional interference knockdown of AβOs by scFvA13-KDEL. (a) On the left, a simplified scheme of the experiment in which the CM from 7PA2 or 7PA2-A13K cells is administered to the primary hippocampal neurons. On the right, WB analysis of ERK1/2, phospho-ERK1/2 (pThr202/pTyr204) and phospho-CREB (pSer133) of the hippocampal neurons treated with 7PA2 CM and 7PA2-A13K CM for 16 h, and histogram of the phosphorylation ratios from densitometric analysis values. Mean values±s.e.m., *P<0.05 Student’st-test,n=3. The 7PA2-A13K CM is effectively depleted of functionally active AβOs by the intrabody-mediated CSI. The modulation of the ERK and CREB signalling pathways by AβOs, mediated by NR2B stimulation, was preliminarily verified by the use of the NR2B-selective antagonist Ro 25-6981 (0.5 μM) (unpublished data) according to the previous reports26. (b) WB (steady-state levels) of mTOR, phospho-mTOR (pSer2448), p70S6K and phospho-p70S6K (pThr389) in 7PA2, 7PA2-A13K and CHO cells and histogram of the p70S6K phosphorylation ratios from densitometric analysis values. Mean values±s.e.m., *P<0.05 Student’st-test,n=3. The scFvA13-KDEL intrabody, through its functional knockdown of AβOs, reduces mTOR activity. Figure 9: Functional interference knockdown of AβOs by scFvA13-KDEL. ( a ) On the left, a simplified scheme of the experiment in which the CM from 7PA2 or 7PA2-A13K cells is administered to the primary hippocampal neurons. On the right, WB analysis of ERK1/2, phospho-ERK1/2 (pThr202/pTyr204) and phospho-CREB (pSer133) of the hippocampal neurons treated with 7PA2 CM and 7PA2-A13K CM for 16 h, and histogram of the phosphorylation ratios from densitometric analysis values. Mean values±s.e.m., * P <0.05 Student’s t -test, n =3. The 7PA2-A13K CM is effectively depleted of functionally active AβOs by the intrabody-mediated CSI. The modulation of the ERK and CREB signalling pathways by AβOs, mediated by NR2B stimulation, was preliminarily verified by the use of the NR2B-selective antagonist Ro 25-6981 (0.5 μM) (unpublished data) according to the previous reports [26] . ( b ) WB (steady-state levels) of mTOR, phospho-mTOR (pSer2448), p70S6K and phospho-p70S6K (pThr389) in 7PA2, 7PA2-A13K and CHO cells and histogram of the p70S6K phosphorylation ratios from densitometric analysis values. Mean values±s.e.m., * P <0.05 Student’s t -test, n =3. The scFvA13-KDEL intrabody, through its functional knockdown of AβOs, reduces mTOR activity. Full size image Furthermore, we reported an independent functional demonstration of the biological relevance of the intrabody-targeted AβO conformers. Indeed, in 7PA2 cells, the activity of mTOR (mammalian target of rapamycin), a crucial mediator of cellular homeostasis and autophagy, is directly linked to the levels of endogenous Aβ [38] . Here, we show that in 7PA2-A13K cells, mTOR activity is reduced back to basal levels (found in CHO cells), as measured by the phosphorylation levels of the direct downstream target p70S6K ( Fig. 9b ). This provides a new functional demonstration that the intracellular AβO conformers targeted by the scFvA13-KDEL are involved in the impaired homeostasis and autophagy in 7PA2 cells, through the mTOR signalling pathway. In conclusion, the functional results, through two independent readouts, demonstrate that both extra- and intracellular pools of AβO conformers targeted by the scFvA13-KDEL intrabody, among the numerous and diverse Aβ and APP-derived soluble species, constitute a crucial pool of active AβOs, directly involved both in the deregulation of specific cellular pathways linked to cellular homeostasis, and in the synaptic actions previously ascribed to the more complex CM of 7PA2 cells, and thought to be relevant in neurodegeneration and also AD pathogenesis. AβOs are considered the most neurotoxic Aβ forms in AD brains, but they are still mysterious entities in terms of molecular and structural composition and activity [8] . Furthermore, while intracellular AβOs are emerging targets in AD studies [7] , [15] , their identification, study and targeting in the complex context of subcellular compartments of living cells still remains a big challenge. This is a key issue, in order to uncover and validate new molecular and cellular targets tightly linked to the Aβ hypothesis, for a successful search and development of novel therapeutics for AD [8] , [39] . While the processes of Aβ aggregation are intensively studied at different levels of complexity ( in silico, in vitro and in vivo ) numberless questions remain open and to be addressed, such as the identification of the cellular mechanisms and the subcellular sites of Aβ misfolding and oligomerization. Of note, in the current state of the art, this question necessarily calls for the development of new selective experimental approaches exploitable in living cells. We face the question in a way not tackled before by establishing a new approach that we called CSI based on the subcellular targeting of a conformation-sensitive intrabody in living cells. In this way, we showed for the first time that it is possible to selectively target, inside the cell, certain oligomeric Aβ conformers but not the Aβ precursor protein (APP) or the monomeric Aβ. This represents a significant advancement with respect to the currently used secretase inhibitors [40] and previous targeting of the Aβ/APP system with intrabodies that were acting through an interference with the processing and/or maturation of APP [41] or of γ-secretase components such as nicastrin [42] . Moreover, the subcellular-localized anti-AβOs CSI, via the retention/retrieval of the KDEL intrabody in the ER, provides significant new insights into the functions of this organelle in the assembly of functionally active AβOs. We show that the main mechanism operated by the ER-resident intrabody is of a conformational assembly modulation, through a mechanism of chaperone-like folding assistance on critical AβO conformers intermediates ( Fig. 10 ). 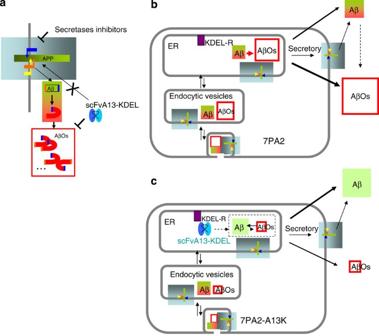Figure 10: Model of mechanism of action of the intrabody-mediated CSI for scFvA13-KDEL. The panels are based on the scheme ofFig. 1brepresenting the APP processing and Aβ generation and oligomerization in the cellular model of APP–RIP used in the study. (a) Proposed mechanism of action of scFvA13-KDEL in the pathway of Aβ generation and assembly: while secretase inhibitors target the APP cleavages, the intrabody controls the assembly of Aβ in pathological AβOs without interfering with the APP processing. (b) Schematic 7PA2 cell used as fAD model of APP–RIP and AβOs generation. Our study demonstrates that the ER is an organelle crucial for the assembly of biologically relevant AβOs. The ER-assembled AβOs are likely the main source of those found extracellularly and they are essential in the intra- and extracellular balance of Aβ and AβO species. (c) In 7PA2-A13K cells, we propose a mechanism by which early-assembled AβO conformers are intercepted by the intrabody in the ER. Thus, the intrabody can be deputed to a selective control of the Aβ misfolding (represented by a change of the green–red-shaded box with a green one) and assembly (represented by smaller red frame boxes in comparison with 7PA2 cells), equipping the ER with new functions of quality control, otherwise escaped by pathological conformations of Aβ. Thus, the main mechanism operated by the ER-resident intrabody is of a conformational assembly modulation. As a consequence, the levels of intra- and extracellular pools of AβOs decrease while secreted Aβ monomers increase. Figure 10: Model of mechanism of action of the intrabody-mediated CSI for scFvA13-KDEL. The panels are based on the scheme of Fig. 1b representing the APP processing and Aβ generation and oligomerization in the cellular model of APP–RIP used in the study. ( a ) Proposed mechanism of action of scFvA13-KDEL in the pathway of Aβ generation and assembly: while secretase inhibitors target the APP cleavages, the intrabody controls the assembly of Aβ in pathological AβOs without interfering with the APP processing. ( b ) Schematic 7PA2 cell used as fAD model of APP–RIP and AβOs generation. Our study demonstrates that the ER is an organelle crucial for the assembly of biologically relevant AβOs. The ER-assembled AβOs are likely the main source of those found extracellularly and they are essential in the intra- and extracellular balance of Aβ and AβO species. ( c ) In 7PA2-A13K cells, we propose a mechanism by which early-assembled AβO conformers are intercepted by the intrabody in the ER. Thus, the intrabody can be deputed to a selective control of the Aβ misfolding (represented by a change of the green–red-shaded box with a green one) and assembly (represented by smaller red frame boxes in comparison with 7PA2 cells), equipping the ER with new functions of quality control, otherwise escaped by pathological conformations of Aβ. Thus, the main mechanism operated by the ER-resident intrabody is of a conformational assembly modulation. As a consequence, the levels of intra- and extracellular pools of AβOs decrease while secreted Aβ monomers increase. Full size image The CSI determines an opposite balance of the different pools of soluble Aβ observed in 7PA2-A13K cells: on one hand, the extracellular LDS/SDS-stable dimers and trimers and the AβO conformers are reduced, and, on the other hand, the extracellular monomeric Aβ peptides are increased, without significant changes in the ratios of Aβ truncated forms. Recent studies show the AD pathological importance of qualitative changes in the γ-secretase-generated Aβ products (species of 37–43 amino-acid length) [43] . Even small changes in the composition of synthetic Aβ mixes can affect critically their aggregation kinetics and toxic effects; in particular, AβOs composed by fAD-like Aβ42:Aβ40 ratios are more stable and toxic [44] . This is in accordance with the differences observed here, between 7PA2 and 7WD4 cells. However, our results in 7PA2-A13K cells (where we observed complementary changes of the secreted AβOs and of Aβ monomers/fragments) additionally show that the ER control of Aβ peptides folding and assembly in vivo , even in the context of their pathological ratios, is a crucial step in the formation of pathologically relevant AβO conformers. In 7PA2-A13K cells, the increased proportion of secreted free monomers can be interpreted as deriving from the intracellular AβO conformers intercepted by the intrabody along oligomerization pathways and representing a fingerprint of their composition (in non-assembled state). Thus, AβOs, when assembled inside the cells and then secreted, would be formed by well-defined ratios of several Aβ peptides and fragments. The Aβ1-42, known to be preferentially generated in the ER [7] , [45] , [46] , could act here as a seed for oligomerization of other Aβ monomers with a mechanism therefore favored by the neutral luminal pH (peculiar of the ER) and by the macromolecular crowding of this organelle. Of note, in vitro studies demonstrate that neutral pH, opposite to acid pH, favors pathways of Aβ oligomerization against fibrillization [47] and that the macromolecular crowding can contribute to the amyloid aggregation [48] . Besides its favourable physicochemical milieu, the ER has a crucial role in the protein quality control and in the physiological oligomerization of some protein complexes, making a priori this organelle a good candidate for our intrabody-targeting study. The chaperone-like mechanism proposed for the scFvA13-KDEL is consistent with the physiological role of ER-resident chaperones engaged in protein folding and/or degradation processes [35] . However, it is unknown if AβOs can be a direct target of endogenous ER chaperones; a study demonstrated that some ER chaperones indirectly regulate the Aβ production through their interaction with APP impairing its maturation and processing [49] . Thus, the scFvA13-KDEL intrabody can equip the ER with new beneficial functions (otherwise lacking in mammalian cells) of selective control of critical AβO assembly. We also surmise that the KDEL system, physiologically exploited by some endogenous ER chaperones for the protein quality control, was likely essential to obtain a chaperone-like action of the intrabody (shuttling between the ER and the Golgi complex). Several studies show that the Aβ peptides can be formed in different subcellular compartments such as ER, Golgi, TGN, endosomes, lysosomes [7] , [34] but no study has been able to address the important question of where and how intracellular Aβ peptides oligomerize. Recently, intracellular AβOs have been identified in fixed cells or brain tissues through oligomeric-specific antibodies, but these antibodies do not allow functional studies of the AβOs formation and trafficking in living cells. Thus, the localization of intracellular AβOs is still an open and controversial question; as for the origin of intracellular AβOs, the prevailing hypothesis suggests the endocytosis of AβOs assembled outside of the cell. However, the extracellular space, such as the extracellular fluid of the brain, is not the ideal milieu for the Aβ aggregation, first due to the very low concentration of soluble Aβ (<1 nM). Accordingly, a study demonstrated that nanomolar concentrations of synthetic Aβ, extracellularly administered to the cultured cells, form amyloid seeds only in the intracellular milieu upon cellular uptake, concentration and aggregation in endocytic vesicles [50] . At difference, our study is performed in living cells where a complex pattern of Aβ peptides is endogenously produced through the APP–RIP occurring in several subcellular compartments. In this context, we recognized the ER as the main and crucial site to control critical events of Aβ oligomerization, just exploiting the precise spatially localized subcellular intrabody probe for CSI (in the ER but not in other endocytic vesicles). However, we cannot exclude that some Aβ oligomerization (or Aβ super assembly onto ER-formed seeding nuclei) could also occur in other subcellular compartments (that is, along the secretory and endocytic pathways), and/or that some Aβ/AβO species can reach the ER through the Golgi complex, during retrograde routes of subcellular vesicular trafficking that is, via the retromer TGN). Finally, we demonstrated that the pool of AβO conformers intercepted in the ER and modulated by the scFvA13-KDEL intrabody is functionally relevant, by exploiting two distinct functional readouts regarding the extrasynaptic activation of ERK/CREB signalling pathways in primary neurons and the phosphorylation pathway of p70S6K, a downstream target of mTOR, implicated in the impaired cellular homeostasis and autophagy. As an interesting parallel to our results, amyloid-binding compounds modulating the Aβ assembly also restored the protein homeostasis during aging in Caenorhabditis elegans models [51] . Given the central role of the ER mitochondria cross-talk in maintaining cellular homeostasis, and given that 7PA2 cells show a prominent set of functional mitochondrial deficits [52] , it will be interesting to investigate whether the scFvA13-KDEL is able to restore normal mitochondrial functions in 7PA2 cells, via its interference with intracellular AβOs in the ER. Our overall results support the idea that targeting specific conformations of Aβ can be a strategy more selective and more effective than lowering its total levels. Furthermore, we show the value of the subcellular targeting for mechanistic studies on Aβ oligomerization in the ER and the early secretory compartment. In addition, intrabodies can be targeted to other subcellular compartments and also to neuronal specialized districts in order to address new relevant questions on different mechanisms of AβOs trafficking and actions. Indeed, the cellular mechanisms of APP processing, Aβ generation and oligomerization can present specific cell-type peculiarities, as in the case of the polarized and specialized neuronal cells. In neurons, APP undergoes fast anterograde transport to nerve terminals and is metabolized within the axonal or presynaptic vesicles into Aβ peptides that are released and deposited as amyloid plaques around nerve terminals [53] , [54] . Furthermore, synaptic activity increases Aβ secretion, indicating that the presynaptic terminal is an important regulatory site for Aβ generation [55] , [56] . Of note, intrabodies can be targeted also to neuronal specialized districts, such as pre- and post-synaptic terminals [57] , [58] . The demonstration of cell-specific (neuronal or not) mechanisms of subcellular AβOs trafficking and actions will be the next goal of our intrabody-based studies, having here established that CSI allows a dissection of AβOs-specific mechanisms not mediated by Aβ monomers nor by APP. In light of the controversial and open questions emerging from Aβ-targeting clinical trials [39] and immunotherapy [59] in AD, we believe that our study provides a new cellular and biochemical basis for targeting AβOs inside cells, and that the CSI approach can be worthy of further preclinical and clinical applications. Of note, the conformation selectivity and the molecular specificity of the CSI approach overcome limits of methods targeting nucleic acid (genes or mRNA) or exploiting new chemical compounds that cannot achieve a comparable molecular and subcellular precision. Finally, the CSI approach can be exploited in different proteinopathies through the upstream direct selection of new functional intrabodies [60] , [61] against antigens that undergo in vivo misfolding, similarly to Aβ [13] . Cell lines 7PA2 and 7WD4 cells (CHO stably transfected respectively with the human APP751 cDNA bearing the V717F fAD mutation and with the wtAPP751, kindly provided by Dr D.J. Selkoe, Harvard Medical School, Boston) were grown in Dulbecco’s modified Eagle’s medium (DMEM) with 10% fetal bovine serum (FBS), 2 mM glutamine and antibiotic selection (G418) as previously described [23] . SHSY5Y human neuroblastoma cells were grown in DMEM-F12 supplemented with 10% FBS and 2 mM glutamine. Intrabody constructs The constructs for scFv-KDEL intrabodies for the ER retention/retrieval, follow the scheme of expression box of the pscFvExpress vector [62] , with an N-terminal SecL, secretory leader sequence from an IgG1 immunoglobulin, and a C-terminal KDEL, ER retention/retrieval signal sequence. A V5 tag is inserted before the C-terminal KDEL sequence and allows the immunodetection of the scFvs, by anti-V5 antibodies. The cDNA of the anti-AβOs scFvA13 (ref. 13 ) (or of the Aβ-unrelated scFvR4 (ref. 63 )) was cloned through the restriction enzyme BssHII-NheI in frame with a C-terminal V5 tag. The secretory construct differs from the KDEL construct only for the lack of the C-terminal KDEL ER retention/retrieval signal sequence. The cDNA of scFvA13 was also cloned in the backbone vector ‘scFv-degradin’ (kind gift of Prof. Burrone, IGEB Trieste) [36] . Establishment of cell lines stably expressing the intrabodies Cells were transfected with scFv-intrabody vectors, coding for scFvA13 or scFvR4, using Lipofectamine 2000 (Invitrogen) and stable cell clones were obtained by limiting dilution in the presence of appropriate antibiotics (250 μg ml −1 G418 and 2.5 μg ml −1 puromycin for 7PA2 and 7WD4 cells, and only G418 for SHSY5Y cells). We established both a polyclonal population and multiple stable single clones. In a preliminary survey, we characterized the levels of intrabody expression (by WB), its subcellular localization (by immunofluorescence) and the modulation of secreted AβOs. Then we performed the overall study on a 7PA2-A13K clone, showing an average expression level and representative of the entire polyclonal population. Cell samples for Aβ/AβOs analyses For CM preparation, cells were grown to ~\n90% confluence, washed twice with Dulbecco’s phosphate-buffered saline (DPBS) and then conditioned in serum-free medium for 18 h. CM was collected and cleared of cell debris by centrifugation at 200 g for 10 min. In comparative analysis of different cell lines, CM was prepared from cells at the same density of plating. The Ponceau S staining of nitrocellulose membrane before WB (detecting the total proteins) and the WB for the extracellular soluble protein Laminin (unpublished data) were used as normalization of WB lanes loading (see also Supplementary Information ). In straight (non-concentrated) 7PA2 CM, Aβ monomers are detectable (by WB and SELDI-TOF MS), while AβOs (by WB and DB) are generally under the detection limits. In order to improve the detection of AβOs (without immunoprecipitation steps), we optimized a procedure of concentration of the CM by centrifugation steps in concentrators with a 3 kDa or a 5 kDa cut-off (VivaSpin Sartorius). We established that a 15 × concentration allows a sensitive discrimination of AβOs (in comparative analyses of 7PA2 and 7PA2-A13K CM). The overall results demonstrate that this procedure is useful to obtain samples, whose concentrations of total Aβ (determined by quantitative WB) are in the range of previous studies, and, most importantly, maintaining the effective conformational-relevant differences of starting non-concentrated samples. Cell lysates were done in Tris-HCl pH8 50 mM, NaCl 150 mM, NP40 1% with the addition of cocktail of proteases and phosphatases inhibitors (Roche). The lysates were centrifuged at 12,000 g for 10 min. The supernatant was collected and the concentration of total proteins was determined by BCA assay. Aβ/AβOs WB analysis Samples (CM or cell lysates) were diluted in 4 × LDS sample buffer, containing reducing agents (DTT or β-mercaptoethanol), boiled 10 min, loaded in precasted Criterion gels XT Bis-Tris 4–12% Bio-Rad, running in MES buffer. The semidry blot was then done onto nitrocellulose membrane filters, 0.22 μm. The membrane filter was boiled in PBS to increase the detection of low MW bands. MAb 6E10 (Covance) or mAb 4G8 (Covance) were used, respectively 1:1,000 or 1:500 in TBS 0.05% tween, 2% dry milk. ECL (GE) chemiluminescent detection was performed. As discussed in the text, the bands at ~\n8 kDa and at ~\n12 kDa correspond to Aβ dimers and Aβ trimers, collectively named LDS/SDS-stable low MW AβOs (due to the analysis method involving LDS in the sample buffer and SDS in the polyacrylamide gel), largely characterized in 7PA2 cells [24] . The identification of the 4, 8 and 12 kDa bands as containing Aβ was confirmed by the use of a γ-secretase inhibitor L-685,458 (ref. 29 ), which almost abolishes the formation of Aβ, and, as a consequence, also of its assemblies, AβOs (see also Supplementary Information ). DB analysis Purified proteins and cellular samples were spotted onto nitrocellulose membrane filters 0.22 μm. The anti-AβOs scFvA13 (3.5 μg ml −1 ) and scFvIm3 (4.5 μg ml −1 ) were used as primary antibodies diluted in TBS 0.05% tween, 5% dry milk with the addition of cocktail of proteases inhibitors (Roche). The polyclonal antibody anti-oligomer A11 (ref. 21 ) was used 1:500 in TBS 0.05% tween, 5% dry milk. The AβO scFv-positive immunodetection was performed by anti-His tag (for cellular samples), or by anti-V5 tag (for monomers and oligomers of synthetic Aβ, α-Synuclein and lysozyme), which respectively recognizes the C-terminal 6xHis tag or V5 tag of recombinant scFvs (expressed in Escherichia coli and purified, see the paragraph below). Serial dilution curves of cellular samples were preliminarily tested to obtain non-saturating condition of immunodetection. Samples were loaded as follows: 450 ng per dot of synthetic human Aβ1-42; 500 ng per dot of recombinant human α-Synuclein; 500 ng per dot of lysozyme; 20 μl per dot of 15 × concentrated 7PA2 CM and related samples (CM of γ-secretase inhibitor-treated 7PA2 cells and 7PA2-A13K CM) by using Bio-Dot SF apparatus Bio-Rad; 500 ng per dot of total lysates (non-denatured). Purified proteins assayed by DB and ELISA Synthetic human Aβ1-42 (HFIP-pretreated peptide, purchased from Anaspec) was dissolved (5 mM) in anhydrous DMSO and assembled to form AβOs as ADDLs (100 μM Aβ in phenol red-free Ham’s F12 medium, purchased from PanBiotech) at 4 °C for 24 h [47] without shaking. Following incubation, tubes were centrifuged at 14,000 g for 10 min in the cold. The supernatant (soluble ADDLs) was recovered and transferred to new tubes, and immediately frozen in dry ice and stored at −80 °C in aliquots of small volume. Several independent ADDLs preparations were assayed by DB and ELISA comprising ADDLs previously prepared and characterized for toxicity and synaptic binding [13] . As Aβ monomers, we used the nonaggregated Aβ1-42 diluted in ice-cold MilliQ water (to a final concentration of 100 μM Aβ) and immediately frozen at −80 °C. Recombinant human α-Synuclein (Abcam), 70 μM in 100 mM NaCl, 20 mM Tris-HCl, 1 mM MgCl 2 (pH 7.5) was sonicated for 10 min in water bath sonicator, aliquoted and immediately frozen at −80 °C or oligomerized by incubating the protein solution at 4 °C for 3 or 7 days without shaking (adapting conditions described [64] ). Purified lysozyme (AppliChem), from chicken egg white, was dissolved in 25 mM KH 2 PO 4 pH 2 at 45 °C, consecutively filtered through 0.22 and 0.1 μm pore size syringe filters and assembled as oligomeric fibrils (0.5 mg ml −1 in 175 mM NaCl/25 mM KH 2 PO 4 pH 2) for 3 h at 50 °C (ref. 65 ); following a different procedure, lysozyme was also dissolved in phosphate buffer (PB) 0.1 M at pH 7.4, filtered through 0.1 μm pore size syringe filters and assembled as oligomers (7 mg ml −1 in PB 0.1 M at pH 7.4) for 4 h at 50 °C (ref. 66 ). The presence of oligomers in the assembled samples was confirmed by ELISA, using as primary antibodies the generic anti-oligomer A11 (ref. 21 ) or the AβO-specific scFvA13 (ref. 13 ) (see also Supplementary Information ). Aβ immunoproteomic SELDI-TOF MS analysis The anti-Aβ mAbs (6E10+4G8, 0.125 mg ml −1 ) (Covance), used as Aβ capturing antibodies, were incubated in a humid chamber for 2 h at room temperature (RT) to allow covalent binding to the PS20 ProteinChip Array (Bio-Rad Laboratories) [27] . Unreacted sites were blocked with Tris-HCl 0.5 M, pH 8 in a humid chamber at RT for 30 min. Each spot was washed first three times with PBS containing 0.5% (v/v) Triton X-100 and then twice with PBS. The spots were coated with 5 μl of sample (CM, straight or 10 × concentrated in a Savant Speed Vac) and incubated in a humid chamber overnight. Each spot was washed first three times with PBS containing 0.1% (v/v) Triton X-100, twice with PBS and finally with deionized water. α-cyano-4-hydroxy cinnamic acid (Bio-Rad) was added 1 μl per spot. Mass identification was made using the ProteinChip SELDI System, Enterprise Edition (Bio-Rad). In comparative studies (7WD4 CM versus 7PA2 CM and 7PA2 CM versus 7PA2-A13K CM), the CM was prepared from cells at the same density of plating; CM was also loaded in polyacrylamide gels, blotted and normalized by Ponceau S staining of nitrocellulose membrane (detecting the total proteins) and analysed by WB as described. Subcellular fractionation Subcellular fractionation on discontinuous iodixanol gradients were made as described [67] . In brief, cells grown to confluence were pelleted and resuspended in homogenization buffer (10 mM HEPES, pH 7.4, 1 mM EDTA and 0.25 M sucrose) supplemented with protease inhibitor cocktail (Roche). Cells were disrupted with a Dounce homogenizer (10 strokes) followed by five passages through a 27-gauge needle. Nuclei and unbroken cells were pelleted and the post-nuclear supernatant centrifuged for 1 h at 65,000 g . The resultant vesicle pellets, nominally total microsomes, were resuspended in 0.8 ml of homogenization buffer. A discontinuous gradient of iodixanol (OptiPrep, Axis-Shield) in 0.25 M sucrose homogenization buffer, was prepared by underlayering with a syringe different density solutions ranging from 2.5 to 30%. The resuspended vesicle fractions were loaded on top of the gradient and centrifuged in a SW40Ti rotor at 40,000 g for 2.5 h (4 °C). The resulting gradient was collected in 12 fractions of 1 ml. Then, each fraction was denaturated and tested by WB for subcellular markers. Intrabody-AβOs co-IP from subcellular fractions Freshly prepared subcellular fractions (or total microsome preparations) were incubated with a cross-linker solution of dithiobis(succinimidyl propionate) (DSP, Pierce), to a final concentration of 2 mM for 30 min at RT, after that Stop Solution (1 M Tris pH 7.5) was added to a final concentration of 20 mM for 15 min. Cross-linked subcellular fractions (or total microsomes) samples were incubated with anti-V5 agarose affinity gel (Sigma) for 16 h at 4 °C for the immunoprecipitation procedure. After ice-cold PBS washes (6 times 5,000 g , 5 min each), the immunoprecipitated proteins were eluted with 4 × Tricine sample buffer (Bio-Rad) containing β-mercaptoethanol by 10 min boiling, electrophoresed on Tris-Tricine gel 16.5% (precasted gels, Bio-Rad). The semidry transfer blot was performed in nitrocellulose membrane filter 0.22 μm and the filter boiled in PBS and subjected to WB analyses (mAb 6E10 anti-Aβ/APP and mAb anti-V5-HRP). Co-IP of small AβOs and intrabody was analysed in Tris-Tricine gels 16.5% for a better resolution of low MWs (<50 kDa) WB bands. The full-length APP (~\n110 kDa) was analysed in Tris-glycine HCl gels 10% or in Criterion Bis-Tris XT Gels 4–12% (Bio-Rad) upon elution and boiling of immunoprecipitated proteins with the appropriate sample buffers (respectively 4 × Laemmli Sample buffer or 4 × XT sample buffer Bio-Rad with β-mercaptoethanol). In vitro assembly interference with synthetic Aβ1-42 The human Aβ1-42 peptide, HFIP-pretreated (Anaspec) was diluted (5 mM) in anhydrous DMSO and then in phenol red-free Ham’s F12 medium (PanBiotech) at 100 μM as previously described [68] . Aliquots were immediately frozen and stored at −80 °C. Before aggregation, 100 μM Aβ1-42 in Ham’s F12 was diluted at 65 μM by adding scFvA13 or NaPB buffer (NaCl 100 mM, sodium phosphate buffer pH7, 20 Mm) as control. The scFvA13 was used at stoichiometric (65 μM) or substoichiometric (13 μM) ratio with Aβ1-42. The aggregation was performed at 22 °C for 24 h. For disassembly assays, stoichiometric (65 μM) or substoichiometric (13 μM) concentrations of the scFvA13 or the NaPB buffer as control were added to Aβ1-42 in Ham’s F12 (preassembled at the concentration of 100 μM, 22 °C for 24 h) obtaining a final concentration of 65 μM Aβ. The disassembly assay was performed at 22 °C for 24 h. Synthetic Aβ samples, not boiled nor treated with reducing agents, were loaded (30 ng per well) in Bis-Tris XT Criterion Gels (Bio-Rad), run in MES buffer and analysed by WB, as described above by 6E10 (Covance), 4G8 (Covance) or by a rabbit mAb anti-Aβ (D54D2, Cell Signalling). ER-localized γ -secretase activity Freshly prepared ER-enriched fractions (from subcellular fractionations) were incubated at 4 °C for determination of basal APP–CTFs and AICD levels, or incubated at 37 °C for 2 h for APP–CTFs γ-secretase cleavage and de novo AICD generation as previously described [31] . Individual fractions were subjected to WB. The detection of AICD was favored by boiling the membrane filter in PBS. BFA treatment Cells (at a confluence of 65–70%) were treated with BFA (10 μM) for 1 or 4 h. After treatment, cells were washed twice with PBS and lysed or were left to recover in fresh growth medium for 2 h before lysis. The lysates were subjected to WB with anti-APP C-terminal antibody (Sigma). Other treatments The γ-secretase inhibitor treatment of 7PA2 cells were performed with 1 μM of L-685,458 (ref. 29 ) (purchased from Calbiochem–Millipore) for 18 h. The proteasome inhibitor MG132 (Sigma) or the inhibitor of protein synthesis cycloheximide (Sigma) was administered at 20 and 40 μM, respectively for 6 h. Hippocampal neuronal cultures Primary rat hippocampal neurons were prepared from embryonic day 18 pups and maintained in vitro in Neurobasal medium with B-27 supplement and 0.5 μM L -glutamine for 14 days (14 DIV). Half the medium was exchanged every 4 days. Neurons (14 DIV) were treated for 16 h with Neurobasal medium conditioned on confluent dishes of 7PA2 cells or 7PA2-A13K cells. Cultures were lysed and subjected to WB, as described [26] . Immunofluorescence analysis Cells were plated on glass coverslips and cultured until reaching ~\n70% confluence, then fixed with 1.9% (v/v) formaldehyde in DPBS (with Ca 2+ and Mg 2+ ) for 5 min, followed by a postfix for 10 min in 3.7% formaldehyde at RT. The coverslips were washed, permeabilized with 0.1% Triton in PBS for 5 min and blocked with 5% FBS in PBS for 1 h at RT. After blocking, cells were incubated with primary antibodies overnight at 4 °C, and then with appropriate secondary antibodies (anti-rabbit or anti-mouse Alexa-Fluor 488 or Alexa-Fluor 594 (Molecular Probes)) for 1 h at RT. Coverslips were mounted with Aqua-Poly/Mount Reagent (Polysciences) and analysed by confocal microscopy. Confocal microscopy Microscopic images were collected at RT using a confocal laser scanning microscope (TCS SP5, Leica Microsystems) equipped with four laser lines and with HCX PL APO lambda blue 63.0 × 1.40 OIL ultraviolet objective. To exclude cross-talk between the emission spectra of fluorophores, images were acquired using the sequential acquisition modality. The acquired images were converted into TIFF files of separated and merged channels by using Leica Application Suite 6000 (LAS AF Lite). Statistical analysis Student’s t -test was used to evaluate differences between two study groups in normally distributed data (two samples, two tails, equal variance). Densitometric analysis WB bands or DB dots images were analysed by using ScionImage software (NIH Image for Windows, Beta 4.0.2). Western Blot analysis Full-lenght images of western blot are shown in Supplementary Figs 14,15 . Preparation of recombinant scFvA13 and scFvIm3 The cDNA of anti-AβOs scFvA13 and scFvIm3 (ref. 13 ) were cloned by restriction with the enzymes BssHII/NheI into the pETM13 vector (modified in the polylinker), and transformed in BL21(DE3)pLysS E. coli (Novagen). The recombinant scFv proteins were prepared following established procedures for the expression and refolding of another SPLINT-derived scFv in the cytoplasm of E. coli [69] . The purification of the refolded scFvs were achieved through a cation exchange chromatography, performed on HiTrap SP column (5 ml, GE), equilibrated with 20 mM sodium phosphate buffer, pH 7 (for scFvA13) and pH 6.5 (for scFvIm3) as A buffer. The elution of the sample was achieved with a linear gradient from 0 to 70% of B buffer (A buffer+1 M NaCl). The sample was then dialysed against PBS and purified on a size exclusion chromatography column, a Superdex 75 (GE), equilibrated with PBS. Antibodies used in WB, DB, IP and immunofluorescence analyses Anti-Aβ/APP 4G8 (mouse mAb, Covance), anti-Aβ/APP 6E10 (mouse mAb, Covance), anti-AβOs scFvA13 and scFvIm3 (ref. 13 ), anti-oligomer A11 (ref. 21 ) (rabbit pAb Millipore), anti-Aβ (rabbit mAb, Cell Signaling), anti α-Synuclein (mouse mAb, Abcam), anti-APP C-terminal fragment (rabbit pAb, Sigma), anti-APP N-terminal 22C11 (mouse mAb, Millipore), anti-V5 (mouse mAb Invitrogen, and rabbit pAb Sigma), anti-V5-HRP (mouse mAb, Sigma), anti-His tag (mouse mAb Millipore), anti-KDEL (mouse mAb, Assay Design/Stressgen) (kind gift of Prof. R. Sitia, HSR San Raffaele, Milan), anti-mTOR (rabbit pAb, Cell Signaling), anti-phospho-mTOR (rabbit pAb, Cell Signaling), anti-P70S6K (rabbit pAb, Cell Signaling) (kind gift of Dr G. Amadoro, CNR, Rome), anti-phospho-P70S6K (rabbit pAb, Cell Signaling), anti ERK1/2 (rabbit pAb, Cell Signaling), anti phosho-ERK1/2 (rabbit pAb, Cell Signaling), anti phospho-CREB (rabbit pAb, Cell Signaling), anti β-Actin (mouse mAb and rabbit pAb, Sigma), anti-calnexin (rabbit pAb, Sigma), anti-GM130 (mouse mAb, Covance), anti-Golgi 58K (mouse mAb, Sigma), anti-Rab3A (mouse mAb, Sigma), anti-Rab5 (rabbit pAb, Abcam), anti-Rab7 (goat pAb, Santa Cruz), anti-TGN46 (rabbit, pAb), anti-LAMP-1 (rabbit pAb, Abcam). Anti-Rab5, anti-Rab7, anti-TGN46 are kind gift of Dr V. Triaca, CNR, Rome. How to cite this article : Meli, G. et al. Conformational targeting of intracellular Aβ oligomers demonstrates their pathological oligomerization inside the endoplasmic reticulum. Nat. Commun. 5:3867 doi: 10.1038/ncomms4867 (2014).